Quantifying through-space charge transfer dynamics in π-coupled molecular systems Understanding the role of intermolecular interaction on through-space charge transfer characteristics in π-stacked molecular systems is central to the rational design of electronic materials. However, a quantitative study of charge transfer in such systems is often difficult because of poor control over molecular morphology. Here we use the core-hole clock implementation of resonant photoemission spectroscopy to study the femtosecond charge-transfer dynamics in cyclophanes, which consist of two precisely stacked π-systems held together by aliphatic chains. We study two systems, [2,2]paracyclophane (22PCP) and [4,4]paracyclophane (44PCP), with inter-ring separations of 3.0 and 4.0 Å, respectively. We find that charge transfer across the π-coupled system of 44PCP is 20 times slower than in 22PCP. We attribute this difference to the decreased inter-ring electronic coupling in 44PCP. These measurements illustrate the use of core-hole clock spectroscopy as a general tool for quantifying through-space coupling in π-stacked systems. Electron transport in conjugated molecules can broadly be characterized as through-space or through-bond in character [1] . Through-space transport is central to many applications of π-stacked systems, such as organic electronics and photovoltaics [2] , [3] , DNA molecular wires [4] , redox active biocomplexes [5] and multilayer graphene devices [6] . Such π-stacked systems are also relevant to single-molecule electronics. For example, strained paracyclophanes have been shown to behave as molecular 'linkers' to connect molecules to metal electrodes in single-molecule circuits [7] . Cyclophanes have also led to a new wave of research into molecular non-linear optical phenomena in donor–acceptor complexes [8] . In the case of organic photovoltaics and light-emitting devices, optimizing the π-stacking of conjugated molecules is essential to tuning transport properties and exciton lifetimes [9] , [10] . Most studies in this field have focused on optimizing bulk device characteristics by altering molecular substituents [11] , post-growth annealing [12] , [13] or other processing steps [14] , or have used scanning tunnelling microscopy and spectroscopy to measure charge transport across multilayer stacks of conjugated molecules [15] . Combined optical absorption spectroscopy experiments and theoretical work on coupling in planar naphthalene dimers has also been published [16] . However, these studies have not provided direct information on charge-delocalization dynamics in these coupled π-systems. In particular, measurements of through-space charge transfer in π-stacked geometries continue to be an experimental challenge [7] . Here we make use of X-ray photoemission spectroscopy (XPS), near-edge X-ray absorption fine-structure spectroscopy (NEXAFS) and the resonant photoemission spectroscopy (RPES) core-hole clock method [17] , [18] , [19] , [20] , [21] , [22] , [23] , [24] , illustrated in Fig. 1a–f , to characterize π–π interaction in conjugated, stacked systems. Core-hole clock spectroscopy has previously been used to measure femtosecond (fs) charge-transfer times between molecule–metal interfaces like C 60 (refs 21 , 25 ), aromatic thiols [26] , [27] , amines [28] and donor–acceptor complexes [29] on Au(111). We now apply this technique to quantify through-space charge transfer from two paracyclophane molecules with distinct intramolecular π-couplings to underlying Au(111) substrates. In large conjugated π-systems, core-level excitons are known to have similar exciton-binding energies and charge density distributions as valence-level excitons [30] . The charge-transfer information gathered by core-level RPES is thus directly applicable to both optically excited and electric field-induced charge transport regimes in these materials. 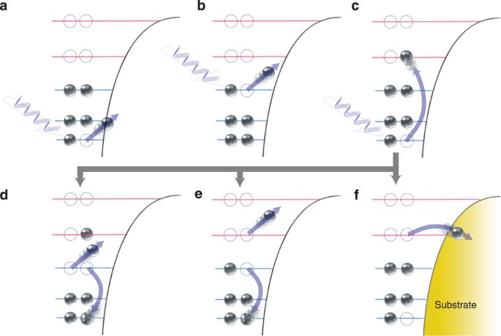Figure 1: Schematic representation of different photoexcitation processes. (a) Direct photoemission from core level (XPS). (b) Direct photoemission from occupied valence states (VB). (c) X-ray absorption-induced transition from core level to lowest unoccupied level; from this excited state, three possible core-hole decay paths are shown. (d) Resonant Auger or spectator decay, (e) resonant photoemission or participator decay and (f) delocalization of excited electron to the unoccupied electronic states of an Au substrate coupled to the molecule. Figure 1: Schematic representation of different photoexcitation processes. ( a ) Direct photoemission from core level (XPS). ( b ) Direct photoemission from occupied valence states (VB). ( c ) X-ray absorption-induced transition from core level to lowest unoccupied level; from this excited state, three possible core-hole decay paths are shown. ( d ) Resonant Auger or spectator decay, ( e ) resonant photoemission or participator decay and ( f ) delocalization of excited electron to the unoccupied electronic states of an Au substrate coupled to the molecule. Full size image We probe the relation between charge transfer dynamics and π–π coupling by comparing two molecules, [2,2]paracyclophane (22PCP) and [4,4]paracyclophane (44PCP), adsorbed on Au(111). 22PCP ( Fig. 2b ) and 44PCP ( Fig. 2a ) can be represented as two benzene rings joined together as eclipsed 'bilayers' using a scaffold of two or four aliphatic carbon chains, respectively. 22PCP is a strained system with an average inter-ring distance of 3.0 Å, whereas 44PCP has an inter-ring separation of 4.0 Å [31] . By comparing these two 'bilayer-like' systems with well-defined, but dissimilar inter-ring distances, we are able to study the effect of inter-ring coupling on through-space charge transport in π-stacked systems [1] , [32] . We find that, despite their very similar interaction with Au(111), the quenching of resonant photoemission processes is stronger in monolayers of 22PCP than in those of 44PCP, indicating a much faster electron delocalization from 22PCP. We develop a model to convert these quenching ratios to charge-transfer times, and are able to distinguish charge transfer from individual rings of each molecule. We find that the charge transfer time across the π-system of 44PCP is about 20 times slower than across that of 22PCP, and attribute this longer charge transfer time to poor through-space coupling between the rings of the molecule. These measurements allow us to quantitatively probe the relation between π–π coupling and charge transfer. 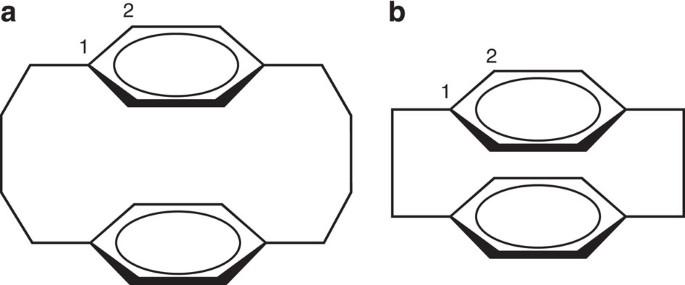Figure 2: Chemical structures. Chemical structures. (a) Chemical structure for [4,4]Paracyclophane (44PCP) and (b) [2,2]Paracyclophane (22PCP). Figure 2: Chemical structures. Chemical structures. ( a ) Chemical structure for [4,4]Paracyclophane (44PCP) and ( b ) [2,2]Paracyclophane (22PCP). Full size image Comparison of monolayer films We first use XPS, NEXAFS and first-principles density function theory calculations to establish that our two systems, 22PCP//Au(111) and 44PCP//Au(111), have similar adsorption configurations, molecule–metal adsorption energies and molecule–metal adsorption distances. 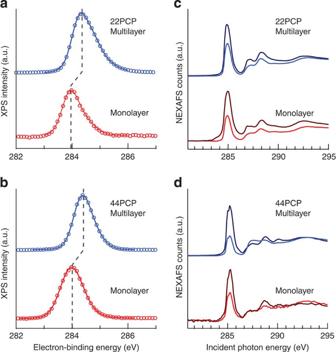Figure 3: XPS and NEXAFS results. (a,b) C1s XPS spectra for 22PCP and 44PCP with multilayer in blue and monolayer in red. Solid lines are fits to data (open circles). (c,d) Carbon K-edge NEXAFS measurements for 22PCP and 44PCP for multilayer (blue) and monolayer (red). The dark (light) blue and red represents incident electric field polarized perpendicular (parallel) to the Au (111) surface. Figure 3a,b show XPS spectra for monolayer and multilayer films of 22PCP and 44PCP. Both molecules show a systematic shift of the carbon 1s (C1s) peak towards higher binding energy with increasing coverage, as expected, due to core-hole screening by the substrate image charge [33] , [34] . We note that both monolayers show the same screening-induced shift to lower binding energy by 0.4 eV relative to the multilayer phase. The C1s peaks for both molecules display similarly broad and asymmetric shapes due to initial state differences between the sp 2 and sp 3 C atoms in the molecules [35] . The similarity in XPS peak positions, shapes and screening-induced shifts for both molecules suggests that there is no large difference in the adsorption energies of the two systems. Temperature desorption spectroscopy shows that both 22PCP and 44PCP monolayers desorb at temperatures between 400 and 420 K, also indicating similar adsorption energies to the Au(111) surface. These experimental findings are corroborated by density function theory calculations for a model system ( Supplementary Methods ), which show that the adsorption energies of 22PCP and 44PCP to an Au-dimer are similar (0.72 and 0.61 eV, respectively) in agreement with previously published results [7] . The optimized adsorption geometries for the dimer–molecule systems are also similar; 22PCP is bound to the dimer at the 1 position, ( Fig. 2 ), with a minimum Au–C bond length of 2.44 Å, whereas 44PCP is bound between the 1 and 2 positions, with a minimum Au–C bond distance of 2.48 Å. These calculations do not reflect the true adsorption energies of these molecules to a Au(111) surface, but do show that no significant difference in the adsorption of 22PCP and 44PCP should be expected. Figure 3: XPS and NEXAFS results. ( a , b ) C1s XPS spectra for 22PCP and 44PCP with multilayer in blue and monolayer in red. Solid lines are fits to data (open circles). ( c , d ) Carbon K-edge NEXAFS measurements for 22PCP and 44PCP for multilayer (blue) and monolayer (red). The dark (light) blue and red represents incident electric field polarized perpendicular (parallel) to the Au (111) surface. Full size image To isolate the effect of inter-ring coupling on charge transfer, it is important to ensure that 22PCP and 44PCP monolayers have similar morphologies on the Au(111) surface. To determine molecular orientation, we carried out NEXAFS dichroism [36] studies on the two systems. Fig. 3c,d show the partial electron yield spectrum collected from the C K-edge of the two samples. To assign peaks, we compared experimental data with simulated NEXAFS spectra using the half core-hole approximation, following Nilsson et al . [37] We found that the sharp feature at 285 eV comprised a doublet, attributed to C1s→π* transitions localized on inequivalent carbon atoms on the benzene rings. The intensity of this peak depends on the orientation of the π* orbital (and thus, the benzene rings) relative to the polarization of incident light. We determine an average tilt angle for the benzene rings with respect to the surface by comparing the ratio of intensities of the peak with incident electric field perpendicular (p-pol) to the sample and parallel (s-pol) to the sample [36] . We find that the average tilt angle for the molecular aromatic rings with respect to the Au(111) surface in monolayer films is 47±5° for 22PCP and 45±5° for 44PCP. This angle is consistent with binding near the 1 or 2 carbon positions on the ring and indicates comparable adsorption geometries for both monolayers. Core-hole clock measurements Having established the adsorption characteristics, we now analyse the charge-transfer characteristics of the two systems via the core-hole clock method. The basic premise of this method is summarized in Fig. 1c–f . Synchrotron radiation is used to induce the transition of a C1s electron to the lowest unoccupied molecular orbital (LUMO; Fig. 1c ), generating an excited electron in the LUMO and a core-hole in the 1s level. In an isolated molecule, such an excited state can decay via one of two processes: a resonant Auger decay, also known as spectator decay ( Fig. 1d ), or resonant photoelectron decay, also known as participator decay ( Fig. 1e ). In either case, a measurable photoelectron intensity results. However, if the molecule is placed on a metal substrate with the LUMO strongly coupled with the metal substrate's wavefunctions ( Fig. 1f ), there is a high probability for the excited electron to delocalize into the continuum electronic states of the metal within the lifetime of the core hole. In this case, both spectator and participator processes are strongly quenched, yielding low or almost no photoelectron intensity. By comparing the intensities of these processes between monolayer and multilayer films of the molecules, we determine a quenching ratio for each molecular system. This quenching can be directly related with the delocalization time for the excited electron, with strong quenching representing fast delocalization. Time resolution of the core-hole clock method is, in principle, limited only by the speed of the clocking process used in the experiment. This method provides information on sub-fs charge-transfer dynamics, which is, to the best of our knowledge, presently inaccessible through other time-resolved spectroscopies [38] . We measure RPES spectra, which comprised XPS measurements taken at a series of incident photon energies across the carbon K absorption edge, on multilayer and monolayer phases of both molecules. Two-dimensional photon energy versus electron-binding energy RPES maps are shown in Fig. 4 . These spectra have been normalized for total Auger intensity. Direct photoemission and Auger electron emission have been subtracted from the RPES images ( Supplementary Methods ), leaving only the photoemission from participator decay. In this figure, we present the region between 284 and 286 eV in photon energy, which contains resonant excitations from C1s to the LUMO and LUMO+1 for both molecules. In both monolayer and multilayer RPES images, high-intensity bands corresponding to these orbital energies are clearly visible. 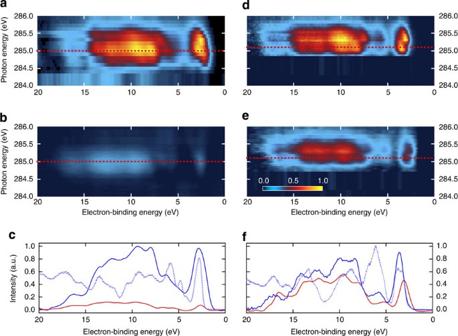Figure 4: Resonant photoemission results. Resonant photoemission (RPES) intensity map of LUMO and LUMO+1 resonances of multilayer (a) and monolayer (b) of 22PCP. (c) Line profiles of LUMO resonances for monolayer (red) and multilayer (blue) 22PCP with the valence band spectrum (dashed blue, 140 eV photon energy). The corresponding panels for 44PCP are shown ind,eandf. The intensities of both valence band spectra have been scaled for clarity. Figure 4: Resonant photoemission results. Resonant photoemission (RPES) intensity map of LUMO and LUMO+1 resonances of multilayer ( a ) and monolayer ( b ) of 22PCP. ( c ) Line profiles of LUMO resonances for monolayer (red) and multilayer (blue) 22PCP with the valence band spectrum (dashed blue, 140 eV photon energy). The corresponding panels for 44PCP are shown in d , e and f . The intensities of both valence band spectra have been scaled for clarity. Full size image Line profiles of the resonant photoemission from the LUMO of 22PCP (285.0 eV) in the multilayer and monolayer phases are taken along the dashed lines in Fig. 4a,b , and are plotted in Fig. 4c together with the multilayer valence band (VB) photoemission spectrum for 44PCP taken separately with a photon energy of 140 eV. Similar profiles are taken for the LUMO of 44PCP (285.1 eV) in Fig. 4d,e , and plotted in Fig. 4f with its VB spectrum. The VB spectra show direct photoemission from the occupied molecular orbitals of each molecule. Each resonant peak in the RPES line profiles corresponds with a peak in the VB spectrum, and thus represents a participator decay process involving distinct occupied–unoccupied orbital pair. It is evident from Fig. 4b,e that the RPES intensity for both molecular monolayers is reduced when compared with the intensity from the corresponding multilayer phases. This decrease in intensity is due to electron transfer from the LUMO to the substrate on a time scale that is comparable to the lifetime of the core hole. The ratio of integrated intensity between monolayer and multilayer films gives us an average quenching ratio, q for each molecular system. For 22PCP, this average quenching ratio q 22 is found to be 0.19±0.02, whereas for 44PCP q 44 is 0.50±0.02, indicating that participator processes in the 22PCP monolayer are strongly suppressed compared with the 44PCP monolayer. As we have shown, the large difference in quenching between 22PCP and 44PCP occurs despite the very similar adsorption characteristics of both molecules on Au(111). Although these quenching ratios suggest that molecule–metal charge transfer from 22PCP is much faster than in 44PCP, we can further quantify the efficiency of charge transfer in each of these π-systems, using a model to convert quenching ratios into charge-transfer times. Using our model, we find that the observed differences in through-space charge transfer between the two molecular systems are a direct consequence of π–π interaction within the molecule. We convert the quenching ratios determined above to overall charge transfer times τ CT using equation (1) below, following the method outlined in ref. 22 : Here, τ CH =6 fs is the core-hole lifetime of C1s [39] , I isolated is the integrated participator intensity from resonant highest occupied molecular orbitals for an isolated molecular system (as approximated by the multilayer) and I coupled is the corresponding intensity for a monolayer film coupled to Au(111). If we simply assume all aromatic carbon atoms in each molecular system to be equally coupled to the substrate (and thus equally quenched), we can calculate an average charge transfer time for each molecular monolayer, τ 22 =1.4±0.5 fs and τ 44 =6.0±0.6 fs for 22PCP and 44PCP, respectively. Within this approximation, our results are consistent with those reported in literature for aromatic molecules adsorbed on metallic substrates. For example, our value of τ 44 =6 fs for 44PCP//Au(111) is the same as that reported for C 60 on Au (110) [40] . Similarly, τ 22 =1.4 fs is within the upper bounds reported for charge transfer times from small, planar aromatics, for example, <3 fs for tetracene on highly ordered pyrolytic graphite (0 0 0 1) [41] . These differences in average charge transfer times provide clues into the relation between through-space charge transfer and inter-ring coupling. But given the symmetries in our system, we are able to go beyond this simple approximation and calculate individual charge-transfer times for the top (further from substrate) and bottom (closer to substrate) rings of these molecules ( Fig. 5a ). We first consider the processes involved during photoemission. As a charge from the C1s core is transferred to the LUMO of the molecule, we compare the calculated LUMOs for both systems with and without a core hole. We see, in Fig. 5b,c , that the ground state LUMO for both molecules is delocalized over both top and bottom rings. However, when a ring atom C1s→LUMO transition occurs, the partially occupied LUMO localizes strongly near the core hole on the same ring ( Fig. 5d,e ) [42] . It is therefore evident that molecule-to-metal charge transfer will depend strongly on the site of the core hole, and excitations in the top ring of a molecule will likely result in slower molecule-to-metal charge transfer than excitations in the bottom ring. Furthermore, comparing Fig. 5d,e , we find that the LUMO in the excited state of 44PCP is much more confined to one ring, which hinders through-space coupling significantly. This comparatively weaker inter-ring coupling in 44PCP results in the lower charge transfer rate we observe. We also note that Fig. 5d,e show that the core hole does not significantly destroy the conjugation within a single aromatic ring. Thus, electronic excitations from any core site on a ring would delocalize very quickly across the LUMO, which is spread across the whole ring. We assume the timescale for this delocalization to be much faster than that of electron delocalization from one ring to another. Thus, the major contribution to differences in charge delocalization is electronic density in between the rings and not differences within a single ring. 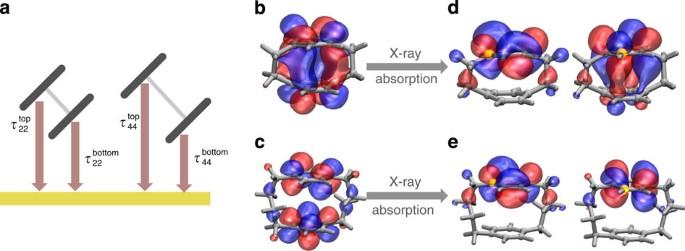Figure 5: Model illustration and calculation results. (a) A schematic of the charge-transfer times calculated by the model. (b,c) Isosurface plots of the ground state LUMO for 22PCP and 44PCP, respectively. (d,e) Isosurface plots for LUMOs in the presence of a core hole for 22PCP and 44PCP. Core-hole excitations on the two inequivalent carbons in the rings (positions 1 and 2 in2) are indicated in yellow. Isosurface values for all plots are set to 0.06 |e|/Å3. Figure 5: Model illustration and calculation results. ( a ) A schematic of the charge-transfer times calculated by the model. ( b , c ) Isosurface plots of the ground state LUMO for 22PCP and 44PCP, respectively. ( d , e ) Isosurface plots for LUMOs in the presence of a core hole for 22PCP and 44PCP. Core-hole excitations on the two inequivalent carbons in the rings (positions 1 and 2 in 2 ) are indicated in yellow. Isosurface values for all plots are set to 0.06 |e|/Å 3 . Full size image To model the charge transfer in these systems, we note that the top and bottom rings of the molecules are simultaneously illuminated, and core holes can be excited in either ring. As we have established that monolayers for 44PCP and 22PCP have similar adsorption geometry, for the rest of this analysis, we assume that the bottom rings of both molecules couple equivalently to the substrate. Therefore, the difference in charge transfer between these two molecules is due to photoexcitation in the inequivalent top rings, where excited electrons must couple across the inter-ring region to delocalize to the substrate. To quantify the above analysis, we develop a one-parameter model for charge-transfer times from top and bottom rings of both monolayers to the substrate (see Methods ). Our model assumes that (1) charge-transfer times from the bottom rings of both 22PCP and 44PCP monolayers are equivalent and (2) charge-transfer times from the bottom rings must be at least as fast as the top rings. With these assumptions, we find that the molecule-to-metal charge transfer from the bottom rings of both molecular monolayers is τ bottom =0.7±0.3 fs, whereas that from the top ring of 22PCP is τ 22 top = 2.3 ± 0.6 fs. We also find that the charge transfer time from the top ring of 44PCP, that is, τ 44 top ≥ 50 fs. An upper bound for τ 44 top would be beyond the experimental limitations of the core-hole clock technique (~10× the core-hole lifetime). Our model shows that charge transfer from the top ring of 22PCP is ~20 times faster than that from 44PCP. We can now compare this measured charge transfer rate difference to the inter-ring coupling in these systems. The molecular orbitals of these compounds can be approximated as bonding and anti-bonding linear combinations of the molecular orbitals of each individual ring (analogous to a xylene). The energy splitting between the bonding and anti-bonding combinations provides a measure of the electronic coupling between the two rings in the ground state. Focussing on the LUMO orbitals, we see that this energy splitting is 1.3 eV for 22PCP compared with 0.21 eV for 44PCP ( Supplementary Fig. S1 ). As the charge-transfer rate is proportional to the square of this energy splitting [43] , we would predict the inter-ring electron transfer rate for 22PCP to be ~40 times higher than that for 44PCP, which is quite close to our experimental result given that we do not include the effect of the underlying substrate or that of the core hole in calculating the coupling. In conclusion, we have determined three distinct charge transfer regimes in paracyclophanes: τ bottom in the sub-fs regime, τ 22 top in the 1–2 fs regime and an extremely long τ 44 top ≥ 50 fs at the experimental limit of the core-hole clock technique. These results present the first measure of through-space charge-transfer time as a function of inter-ring distance in a π-stacked system. By our choice of molecules, and our experimental and theoretical analysis, we are able to quantitatively relate these charge-transfer times to π–π coupling by controlling both inter-ring distance (and hence coupling) and the interaction of molecule to metal. In particular, in the case of extended π-conjugated systems, this quantitative understanding of charge dynamics from core-level spectroscopy can directly be translated to valence exciton dynamics that are relevant to organic photovoltaics and organic light-emitting diodes operating in the visible spectrum [30] . We therefore consider our methods, model and results with cyclophanes to be generalizable to many other π-stacked materials to probe both intra- and intermolecular charge transfer. Experimental methods Our experiments were conducted on the ALOISA/HASPES beamline at the Elettra Synchrotron in Trieste, Italy [44] , [45] , [46] . The Au(111) substrate was first cleaned using a 1 keV beam of Ar 1+ from a sputtering source, followed by a rapid anneal to 900 K. Reflection high-energy electron diffraction was then used to confirm the characteristic herringbone reconstruction of Au(111). XPS measurements were made to ensure no contamination on the sample. The operational pressure for the measurement chamber was maintained at 10 −11 mbar and the sample preparation chamber was maintained at 10 −10 mbar. Both 22PCP and 44PCP were obtained in powder form from Sigma-Aldrich (>97% purity) and used without further purification. Deposition techniques for both molecules were similar. The molecule was placed in a valved, quartz Knudsen-type cell in line-of-sight with the sample preparation chamber. For monolayer deposition, the Au(111) substrate was maintained at room temperature, and the Knudsen cell was heated to 340 K. The molecules were deposited at a chamber pressure of 10 −8 mbar for 3 min. Maintaining the substrate at room temperature during deposition resulted in a monolayer film for both compounds, as determined by Helium angle scattering and XPS measurements. After the chamber recovered to base pressure, the sample was cooled to 230 K before exposure to synchrotron radiation to avoid beam-induced damage. For multilayer deposition, the substrate was first cooled to 230 K, and molecules were deposited at 10 −8 mbar for 5 min. Multilayer films created this way were at least 2 nm thick. After each deposition, XPS spectra of oxygen 1s and nitrogen 1s were checked to ensure no contamination. The films were then characterized using XPS, VB spectroscopy and NEXAFS before conducting RPES measurements. For XPS measurements ( Fig. 3a,b ), X-rays with electric field perpendicular to the sample (p-pol) of energy 400 eV (22PCP) and 500 eV (44PCP) were used at grazing incidence (4 o ) to the sample. Photoelectrons were collected normal to the sample using a hemispherical electron analyser with an acceptance angle of 1 o . The energy scale for XPS spectra was calibrated by aligning the Au 4f 7/2 peak to a binding energy of 84 eV. VB measurements were also carried out under similar beam conditions, except at an incident energy of 140 eV. NEXAFS measurements were conducted on the C K-edge, with incident photon energy between 280 and 295 eV, and incidence angle of 6 o . Spectra were acquired in partial electron-yield mode, with a high-pass filter set to 250 eV and normalized to the beam current measured on the last aperture of the beam path. The spectra were collected with electric-field polarization parallel to the sample (s-pol) and perpendicular (p-pol) to the sample ( Fig. 3c,d ). RPES was conducted by taking XPS scans at a series of incident photon energies between 280 and 295 eV. The sample was moved to a new position after each XPS measurement to ensure that the entire RPES spectrum was taken on a fresh sample. For all RPES measurements presented in this study, incident light was polarized at 54.7 o with respect to the surface normal, which resulted in an RPES signal independent of molecular orientation [36] . The electron analyser for RPES was placed at 54.7 o from the surface normal and along the photon electric field. Charge-transfer model Charge-transfer times from the top rings of both 22PCP and 44PCP monolayers are determined using a one-parameter model, assuming that the bottom rings of both monolayers couple equivalently to the underlying substrate. This assumption is validated by our experimental results, which find similar adsorption energies and geometries of both monolayers on Au(111). The molecule-to-metal charge-transfer time for the bottom rings is thus taken to be equal: To apply equation (1), we must also know the participator intensity contributions from top and bottom rings of the monolayers without charge transfer processes. The top and bottom rings should each contribute half of the measured participator intensity, I isolated mono . However, electrons emitted from the bottom ring can scatter inelastically from the top ring, decreasing the effective contribution from the bottom ring to 0.475 ( Supplementary Methods ). Applying equation (1), we get: where I coupled bottom is the participator intensity for a coupled monolayer due to the bottom ring, I coupled bottom is the corresponding intensity for an uncoupled monolayer and q bottom = I coupled bottom / I isolated mono is the quenching ratio due to charge transfer from the bottom ring to the substrate. A similar procedure is applied to calculate τ 22 top and τ 44 top , the charge transfer times from the top rings of 22PCP and 44PCP: where q 22 and q 44 are the average quenching ratios for 22PCP and 44PCP (as defined in the Results section). The only free parameter within this model is q bottom , the quenching due to charge transfer from the bottom ring to the substrate. We establish bounds for this value by noting that 0 < τ bottom ≤ τ 22 top ,τ 44 top , that is, charge transfer from the bottom ring must be faster than from the top rings. How to cite this article: Batra, A. et al . Quantifying through-space charge transfer dynamics in π-coupled molecular systems. Nat. Commun. 3:1086 doi: 10.1038/ncomms2083 (2012).